Quantum oscillations from surface Fermi arcs in Weyl and Dirac semimetals In a magnetic field, electrons in metals repeatedly traverse closed magnetic orbits around the Fermi surface. The resulting oscillations in the density of states enable powerful experimental techniques for measuring a metal’s Fermi surface structure. On the other hand, the surface states of Weyl semimetals consist of disjoint, open Fermi arcs raising the question of whether they can be observed by standard quantum oscillatory techniques. Here, we find that the open Fermi arcs participate in unusual closed magnetic orbits by traversing the bulk of the sample to connect opposite surfaces. These orbits have anomalous features that are impossible for conventional surface states, and result in quantum oscillations that contain observable signatures of the topological character of the bulk Weyl semimetal. We also apply our predictions to the compounds Cd 3 As 2 and Na 3 Bi that were recently proposed to be three-dimensional Dirac (doubled Weyl) semimetals, and propose experimental signatures of their possible Fermi arc states. Weyl semimetals (SMs) are three-dimensional materials for which the bulk bandgap closes at an even number of discrete points (Weyl nodes) in the Brillouin zone [2] , [3] . Near the Weyl nodes, electrons have relativistic dispersion ε k ≈± υ | k |. Each Weyl node acts as a monopole or anti-monopole of Berry curvature (that is, a closed surface in momentum space surrounding a node will be pierced by ±2 π Berry flux) and is associated with a positive or negative chirality, respectively. Consequently, two-dimensional (2D) cross sections of the Brillouin zone change Chern number by ±1 across each Weyl node, implying that a generic surface will exhibit surface states whose Fermi surfaces consist of a set of open line-segments [2] , [3] , [4] . These Fermi arcs connect pairs of bulk Weyl nodes with opposite chiralities and cannot be removed without annihilating the bulk Weyl nodes. Such unusual surface Fermiology would be impossible in a purely 2D system, whose Fermi surface is necessarily smooth, and cannot abruptly terminate at a point within the Brillouin zone. Consequently, the Fermi arcs serve as a surface fingerprint of the topological character of the bulk band structure, and it is interesting to ask how they might be experimentally observed. Traditionally, the most powerful methods of mapping out a material’s Fermi surface rely on periodic-in-1/ B quantum oscillations of the density of states in a magnetic field, B . Such quantum oscillations require closed magnetic orbits for electrons at the Fermi surface, which naively cannot arise from disjointed Fermi arcs. This raises the interesting question: do Fermi arcs lead to quantum oscillations? We answer this question in the affirmative by noting that, in a slab of Weyl SM of finite thickness, closed magnetic orbits can be obtained by traversing the Fermi arc on the top surface and returning along the corresponding arc on the bottom surface. Using semiclassical methods, we find that such closed orbits can indeed lead to periodic-in-1/ B quantum oscillations of the density of states. Since the orbits involved require an electron to traverse the bulk to connect top and bottom surfaces, the oscillations only occur up to a critical field strength, which depends on slab thickness. For larger fields, the orbits no longer produce periodic quantum oscillations, but are important for understanding the fate of the bulk chiral Landau levels (LLs) and associated chiral anomaly in finite systems. The semiclassical results are then validated by direct numerical simulation of the spectrum of a Weyl SM slab in a field. Weyl SMs are theoretically predicted to occur in strongly spin–orbit coupled systems like the iridates, certain spinels and topological insulator (TI)–ferromagnet multilayers [2] , [5] , [6] , [7] . Yet, despite promising indications [8] , there is currently no clear-cut experimental candidate. However, two recently discovered materials Cd 3 As 2 (refs 8 , 9 , 10 ) and Na 3 Bi [12] , [13] , [14] are thought to be three-dimensional Dirac SMs [15] , close cousins of Weyl SMs. The bulk band structure of these Dirac SMs consists of two superimposed copies of Weyl SMs with opposite chiralities. Ordinarily, when Weyl nodes of opposite chirality are not separated in momentum, they can mix and gap each other out. However, in Dirac SMs, intermixing is symmetry forbidden, since the superimposed Weyl nodes belong to different representations of the crystal symmetry (namely, discrete screw symmetries for Cd 3 As 2 and Na 3 Bi (refs 10 , 11 , 12 , 13 )). We show that the known Dirac SM materials can have pairs of surface arcs that meet at a sharp corner or ‘kink’ at the bulk Dirac nodes. Such a kink would not be allowed in a purely 2D metal, and is a special feature of the crystal symmetry-protected Weyl structure of the Dirac SM. This result is not a priori obvious since the surfaces of interest do not preserve the symmetry that protects the bulk Dirac nodes. Despite this, we show that surface states and kink feature are perturbatively stable to the symmetry-breaking potential of the surface, and can exist so long as this potential is not too strong. Applying the semiclassical results for the Weyl SM, we describe the signatures of these unconventional Dirac surface states in quantum oscillations experiments. Semiclassical analysis To start, let us consider the simplest case of a single pair of bulk Weyl nodes with chiralities ±1 located at k =± k W and a magnetic field B along the y direction (the extension to more complicated cases is straightforward). In an infinite system, the magnetic field produces LL bands that disperse only along the field direction. For k W ℓ B >>1, where is the magnetic length, the ±-chirality Weyl nodes are effectively decoupled, and the LL spectrum includes gapped, non-chiral LL bands with energies with n =1, 2, … and gapless chiral modes with energies , for the ±-chirality nodes, respectively. Now consider a slab of Weyl SM that is infinite in the - and -directions and with finite thickness, L , along ŷ . Further, suppose that the slab is sufficiently thick to neglect direct tunnelling between states in the centre of the Fermi arcs on the top and bottom surfaces. Initially, we focus at low energies near the bulk Weyl node where the relevant states are those of the surface Fermi arc and the bulk chiral LLs. Later, we will see that the results extend to energies well above the Weyl node where the bulk consists of two Fermi pockets connected at the surface by Fermi arcs [4] . In a semiclassical description, an electron at z momentum k z along the Fermi arc of the top surface slides along the arc towards the ‘−’ chirality Weyl node according to: Here we have taken the velocity, υ , on the Fermi arc to be independent of k , and is the unit tangent vector to the arc (with orientation on top and bottom surfaces indicated by the arrows in Fig. 1a ). As an electron sliding along the top-surface arc nears the ‘−’ bulk Weyl node, the energy gap to bulk bands vanishes. This necessarily leads to breakdown in the single-band semiclassical description in which the electron is transferred from the surface arc into the bulk ( Supplementary Note 2 ). At low energies, the only available bulk states are those of the gapless bulk chiral LL [2] ( Fig. 1b ) propagating towards the bottom surface. This chiral mode acts as a one-way ‘conveyor-belt’, transporting the electron from the Fermi arc on the top surface to that of the bottom surface. On reaching the bottom-surface Fermi arc, the electron then slides to the ‘+’ Weyl node, where it connects with the upwards moving chiral bulk LL, thereby returning to the top surface and completing the orbit (see Fig. 1c ). 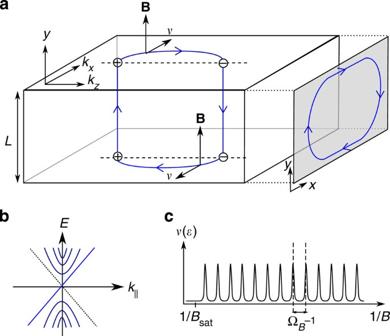Figure 1: Quantum oscillations from Weyl Fermi Arcs. (a) Semiclassical orbit in a magnetic field alongŷ, involving surface states that gives rise to quantum oscillations in a finite thickness slab (shown in mixed real space inyand momentum space inx,zdirections; inset shows corresponding real-space trajectory); (b) bulk LL spectrum for a ‘+’chirality Weyl node,k∥denotes momentum along the direction of the field; (c) periodic-in-1/Bfeatures in the density of states resulting from quantizing the orbits shown in (a). The train of peaks ends at a saturation fieldBsat, which scales inversely with the sample thicknessL. Figure 1: Quantum oscillations from Weyl Fermi Arcs. ( a ) Semiclassical orbit in a magnetic field along ŷ , involving surface states that gives rise to quantum oscillations in a finite thickness slab (shown in mixed real space in y and momentum space in x , z directions; inset shows corresponding real-space trajectory); ( b ) bulk LL spectrum for a ‘+’chirality Weyl node, k ∥ denotes momentum along the direction of the field; ( c ) periodic-in-1/ B features in the density of states resulting from quantizing the orbits shown in ( a ). The train of peaks ends at a saturation field B sat , which scales inversely with the sample thickness L . Full size image Quantum energy levels can be approximately obtained from semiclassical orbits that satisfy the condition: ε n t ≈2 π ( n + γ ) with n εZ, where t is the semiclassical time associated with the orbit, and γ is a constant of order unity encoding low- n quantum effects. Sliding along the top and bottom Fermi arcs takes time: where k 0 is the arc length of the Fermi arc (generally k 0 ≳ k W , the linear distance between bulk Weyl nodes, due to non-zero curvature of the arc). Propagation between top and bottom surfaces via the bulk chiral LL’s takes time . Combining these expressions gives: where zero energy corresponds to the Weyl nodes. These magnetic orbits involving Fermi arcs are distinguished from conventional magnetic orbits in ordinary 2D systems or in surface states of three-dimensional systems by the dependence on the slab thickness, L . As explained below, this characteristic L dependence can be extracted by analysing the dependence of quantum oscillations on field direction. Another peculiar and unconventional feature is that the real-space trajectory of these orbits need not enclose any area perpendicular to the magnetic field (as occurs when the Fermi arcs are straight lines). Quantum oscillations Having established the existence of quantized magnetic orbits involving Fermi arcs, we now turn to the question of whether these orbits produce quantum oscillations. Suppose we fix the chemical potential, μ , and vary magnetic field, B . Equation (2) dictates that the n th energy level crosses μ when: where the solution is defined only for sufficiently large n such that the right-hand side is positive. States cross μ at regularly spaced intervals in of size . Each time a level passes through μ , a peak occurs in the density of states, giving rise to periodic-in-1/ B oscillations in many measurable quantities like conductivity and magnetization. These oscillations are analogous to those of an ordinary 2D metal with quadratic dispersion with effective mass (though, of course, the bulk Weyl electrons are massless and m eff is just an effective parameter with dimensions of mass), and momentum space area A eff =2 k 0 μ / υ . The periodic train of peaks persists only up to fields of order where ⌈ x ⌉ denotes the smallest integer that exceeds x . For fields of order a few Tesla, ℓ B ≈10’s of nm, whereas k 0 is expected to be an atomic scale distance of order 0.1 Å −1 . Hence, quantum oscillations should be observable in slabs a few hundred nm, not too stringent a requirement. Another practical issue is that of impurities. Observation of coherent quantum oscillations requires electrons to complete a magnetic orbit before scattering off an impurity: ω c τ >>1 where and τ is the elastic scattering time. Together with the condition that B < B sat , this requires that the sample thickness does not greatly exceed the mean-free path: . We note that in high-mobility materials, like the Dirac SM candidate Cd 3 As 2 , mean-free paths can be a several hundred nm long in which case L ≪ ℓ is not a stringent condition. For B > B sat , the majority of the magnetic orbit takes place in the bulk, and the energy levels saturate to the field independent values: . Since, the bulk level structure of a thermodynamically thick slab cannot depend on particular choice of boundary conditions, to understand this result, it is useful to compare with a large system with periodic boundary conditions in y . There we expect two sets of B -independent energy modes associated with the ± bulk chiral LL’s, each with quantized energies . The factor of two difference between the quantization scale periodic and open boundary conditions can be understood as follows: in the periodic boundary-condition case, the chiral LL’s from the ± Weyl nodes are independent leading to a doubly degenerate tower of modes. In the finite slab, the ± chiral LL’s are no longer separately quantized, since an electron propagating in the ‘+’ Weyl nodes necessarily reflects into the counter-propagating chiral LL of the ‘−’ Weyl node via a detour through the surface states. However, in the L →∞ limit, such distinctions become unimportant. Distinguishing surface and bulk contributions As essential ingredients for the existence of bulk chiral LLs in a thick but finite slab, these magnetic orbits must persist to all energies where the bulk chiral LLs are present, even when bulk Weyl nodes are doped to form two Fermi pockets. This expectation is indeed borne out by numerical simulations (see below and Supplementary Note 3 ). We now describe how surface and bulk contributions can be distinguished in a doped Weyl SM. For chemical potential, μ , below the first bulk LL, , only surface arcs contribute to quantum oscillations. For higher doping where the bulk FS consists of two disconnected pockets, the surface arc contribution coexists with bulk quantum oscillations. The surface and bulk contributions can be separated due to their different periodicity (see Supplementary Fig. 2 ). In surface-sensitive probes like tunnelling, both have similar magnitudes and the surface oscillations can readily be isolated. For bulk-sensitive probes like magnetization or conductivity, surface arc oscillations may be obscured by the bulk signal in thick or highly doped samples. In fact, contrasting surface and bulk-sensitive probes could directly confirm the surface character of the arc oscillations. The ratio of bulk to surface amplitudes for a slab of thickness L is roughly given by the ratio of bulk to 2D surface density of states (we note for a Weyl SM ). Hence, to directly detect surface arc oscillations with bulk measurements, the bulk contributions can be suppressed by reducing either doping or film thickness. Direction dependence of field So far, we have considered field along the y direction, normal to the surface. For generic field direction B , the bulk chiral LL’s propagate parallel to the field, and only the y component of B drives motion of k along the arc. Ignoring the arc curvature, one can then simply replace and inequations (2) and (3). Notably, the field-scales of equation (3) extrapolate to the residual n =0 value: . The constant piece, eL / k 0 , encodes the deviation of the orbit from a purely 2D orbit and can be extracted by fitting the angle or energy dependence. Deviations from adiabaticity In the above treatment, we assumed that electrons slide all the way to the end of the surface arc before transitioning into the bulk. A more careful analysis ( Supplementary Note 2 and Supplementary Fig. 1 ) shows that the electron jumps off the arc before reaching the end when its momentum is within of the bulk Weyl node. This amounts to replacing in equation (2), where is a numerical constant of order unity. This effect is negligible at low fields k 0 ℓ B ≫ 1, and gives a fractional correction in the quantum oscillation period for high fields. The high-field stretching of is maximal near B ≈ B sat where . Numerical validation of semiclassical approximations We validate the semiclassical treatment by directly obtaining the spectrum of a Weyl SM slab in a magnetic field. Representative results are shown in Fig. 2 . 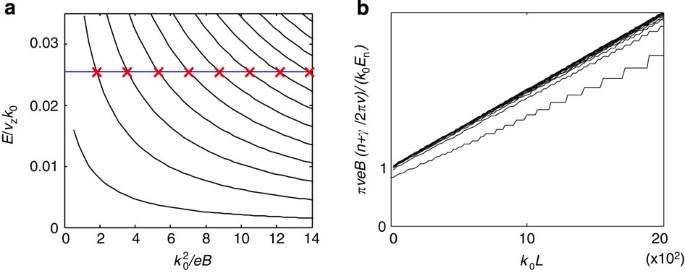Figure 2: Numerical simulations of Weyl slab in a magnetic field. Energy levels with partial surface-bound state character, obtained from numerical solution of equation (4). (a) showsof energy levels with parametersk0L=15 andυ⊥=0.2υz. The levels cross (red crosses) a fixed reference energy (horizontal blue line), with nearly equal spacing for(corresponding to periodic-in-1/Bquantum oscillations), then stop crossing for. (a) (corresponding toB≈1 T for typical expected value ofk0≈0.1 Å−1). (b) shows thatn>0 levels collapse to expected semiclassical form. Only the lowest energy level deviates from the expected semiclassical form, (the jaggedness of this line is a numerical artifact). Figure 2a shows the magnetic field dependence of energy levels corresponding to mixed surface/bulk orbits, and their intercept with a line of fixed energy as a function of inverse-field. The crossings are regularly spaced for small fields, and saturate to B -independent values at large fields. For moderate fields, we observe the predicted stretching of the , due to departures from adiabaticity ( Supplementary Note 2 ). Moreover, when plotted as a function of slab thickness, L , the energy levels ε n collapse to the predicted semiclassical form of equation (2) ( Fig. 2b ). The good agreement with numerics validates the semiclassical approach, which we now extend to treat quantum oscillations from surface states in Dirac materials. Figure 2: Numerical simulations of Weyl slab in a magnetic field. Energy levels with partial surface-bound state character, obtained from numerical solution of equation (4). ( a ) shows of energy levels with parameters k 0 L =15 and υ ⊥ =0.2 υ z . The levels cross (red crosses) a fixed reference energy (horizontal blue line), with nearly equal spacing for (corresponding to periodic-in-1/ B quantum oscillations), then stop crossing for . ( a ) (corresponding to B ≈1 T for typical expected value of k 0 ≈0.1 Å −1 ). ( b ) shows that n >0 levels collapse to expected semiclassical form. Only the lowest energy level deviates from the expected semiclassical form, (the jaggedness of this line is a numerical artifact). Full size image Quantum oscillations from Dirac surface arcs Dirac SMs consist of two superposed copies of a Weyl SM, denoted R and R′ , which transform differently under crystal symmetry preventing them from mixing. Viewed as a doubled Weyl SM, one expects Dirac SM surfaces to exhibit two sets of Fermi arcs that generically curve in opposite directions, and join at the bulk Weyl nodes without mixing ( Fig. 3a,b ). This results in a sharp corner or ‘kink’ in the shape of the surface states’ Fermi surface ( Fig. 3b ). Such a kink would not be allowed in a purely 2D metal, and is a special feature of the crystal symmetry-protected Weyl structure of the Dirac SM. 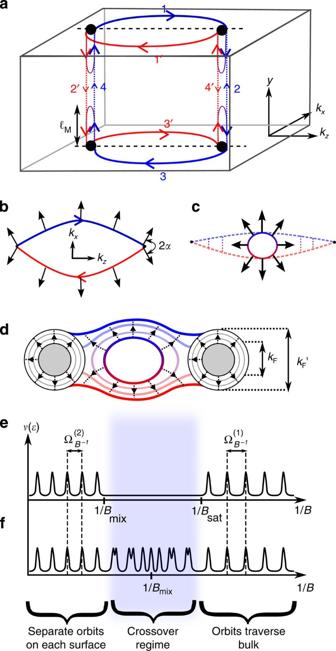Figure 3: Surface states and quantum oscillations in Dirac SMs. Viewing the Dirac SM as two superposed copies of a Weyl SM with opposite chiralities suggests two sets of surface arcs, labelledR(blue) andR′ (red), that curve in opposite directions and meet at the bulk Weyl nodes with a discontinuous kink (a,b). Crystal symmetry-breaking perturbations mixRandR′, but the corner/‘kink’ feature in (b) is perturbatively stable against this effect (vertical dashed lines). A sufficiently strong surface potential may reconstruct the surface arcs into a ‘conventional’ surface state (c), but cannot remove it entirely due to bulk topological contraints. Then for sufficient bulk doping, a surface state initially near the Γ point will intersect the bulk Fermi pockets as shown in (d) for two different bulk Fermi wavevectorskFand. The surface states exhibit spin–momentum locking as indicated schematically by the small black arrows in (b–d). Strong magnetic fields mix theRandR' chiral LLs in the bulk, and lead to a crossover from magnetic orbits through the bulk at low fields to orbits confined near each surface at high fields with two possible intermediate crossover behaviours (e,f). Figure 3: Surface states and quantum oscillations in Dirac SMs. Viewing the Dirac SM as two superposed copies of a Weyl SM with opposite chiralities suggests two sets of surface arcs, labelled R (blue) and R ′ (red), that curve in opposite directions and meet at the bulk Weyl nodes with a discontinuous kink ( a , b ). Crystal symmetry-breaking perturbations mix R and R ′, but the corner/‘kink’ feature in ( b ) is perturbatively stable against this effect (vertical dashed lines). A sufficiently strong surface potential may reconstruct the surface arcs into a ‘conventional’ surface state ( c ), but cannot remove it entirely due to bulk topological contraints. Then for sufficient bulk doping, a surface state initially near the Γ point will intersect the bulk Fermi pockets as shown in ( d ) for two different bulk Fermi wavevectors k F and . The surface states exhibit spin–momentum locking as indicated schematically by the small black arrows in ( b – d ). Strong magnetic fields mix the R and R ' chiral LLs in the bulk, and lead to a crossover from magnetic orbits through the bulk at low fields to orbits confined near each surface at high fields with two possible intermediate crossover behaviours ( e , f ). Full size image Then, in a magnetic field normal to the surface, one expects two sets of energy levels corresponding to the unconventional magnetic orbits described above. Exactly as for the Weyl case described above, these two sets of orbits would produce quantum oscillations for fields below , and the non-trivial mixed surface-bulk character of these magnetic orbits can be observed by extrapolating 1/ B n to n =0 and extracting the angle and chemical potential independent piece . In the remain sections, we show that such doubled Weyl arc type quantum oscillations can indeed occur. However, there are additional complications that must be considered. Effects of reduced symmetry at the surface The first such complication is that, in Cd 3 As 2 and Na 3 Bi, the bulk Dirac nodes are protected by a discrete rotation symmetry around the axis connecting the bulk nodes. This symmetry is broken at all surfaces that could host Fermi arcs (that is, surfaces for which the bulk Dirac nodes project on to different points, leaving room for Fermi arcs to connect them). Hence, the R and R ′ Fermi arcs can hybridize at the surface. Naively, this would immediately gap out the sharp ‘kink’ feature resulting in conventional surface states. However, this is not the case, since where the arcs approach each other at the bulk Dirac nodes, the arc wave functions spread into the bulk where the crystal symmetry is intact. In Supplementary Note 4 , we show that the ‘kink’ feature is perturbatively stable to the symmetry-breaking potential of the surface. Hence when this potential is not too strong, the surface arcs survive and their Fermi surface retains the unconventional ‘kink’ discontinuity. In this regime, one can observe doubled copies of the Weyl quantum oscillations described above (see, however, the subsequent section on the symmetry-breaking effects of the magnetic field). On the other hand, a sufficiently strong surface potential can destroy the sharp corner, resulting in ‘conventional’ (see, however, the discussion in the following section) 2D surface states ( Fig. 3c ). However, as we will now show, for Cd 3 As 2 and Na 3 Bi, there is a non-trivial bulk topological structure which guarantees the existence of an odd number of non-degenerate surface states. Hence, the surface symmetry breaking cannot entirely remove the surface states. Bulk topology and its implications for surface states The Dirac SM materials Cd 3 As 2 and Na 3 Bi can be obtained from a trivial insulator by inverting s - and p - bands with opposite parity eigenvalues at the Γ point. This inversion results in a surface of band crossings where the bands hybridize producing a gap everywhere except along the high-symmetry axis , resulting in two Dirac points. Suppose we weakly break the axial crystal symmetry, this makes each Dirac point massive, producing a full bandgap at the Fermi level and the system becomes a strong TI [10] , [15] , [16] . Importantly, the system becomes a TI regardless of the type of Dirac mass introduced so long as time-reversal (TR) symmetry is preserved and the Dirac points remain at generic non-time-reversal invariant momenta (TRIM) points in the bulk Brillouin zone. This is easiest to see in the presence of inversion symmetry, where the strong TI topological invariant depends only on parity eigenvalues at TRIMs [17] , and cannot be effected by perturbations to the Dirac nodes that occur at generic points in the Brillouin zone. Alternatively, the Dirac mass of each Dirac cone can be parameterized by an axion angle θ , which appears in a magnetoelectric term [18] in the presence of electric and magnetic field E and B . Since θ is odd under TR and the two Dirac nodes are related by TR, any TR invariant Dirac masses satisfying the discussed conditions give cancelling contributions to the total θ angle of the system and cannot change the system from a TI with θ tot = π to a trivial one with θ tot =0. Hence, at the surface of Cd 3 As 2 and Na 3 Bi with a weak bulk crystal symmetry-breaking perturbation, there are an odd number of non-degenerate (that is, spin–momentum locked) surface states. If we then restore the bulk rotation symmetry, the topological surface state cannot be removed by deforming it inside the bulk node without breaking TR symmetry (so long as the Dirac points occur at generic non-TRIM points). This is an interesting new example of symmetry-protected topology in a zero-bandgap system. A novel feature of the surface arcs in scenario Fig. 3a , is that the surface-state Berry curvature is no longer precisely quantized to π . Rather, a non-universal amount of Berry curvature can be ‘hidden’ inside the bulk node as illustrated in Fig. 3b . Such topological features of Dirac SMs are also discussed in ref. 16 . The bulk topology constrains the possible surface state structures. Interestingly, if the scenario shown in Fig. 3c is realized at zero doping, then at some finite doping before the bulk, Fermi pockets merge into a single Fermi sea, the surface arcs will interesect the bulk Fermi pockets (see Fig. 3d ) and enable the quantum oscillations described above. Reduced symmetry in a magnetic field A final complication to viewing the quantum oscillations of Dirac surface arcs as two copies of those of a Weyl SM is that, for Cd 3 As 2 and Na 3 Bi, an applied magnetic field along any axis besides z —breaks the discrete rotation symmetry protecting the Dirac nodes. Consequently, the bulk chiral LLs for the two sets of overlapping Weyl nodes are mixed by the field, and develop a gap , where C is a material parameter ( Supplementary Note 5 ). Henceforth, we will refer to this effect as RR ′-mixing. States with energies ε >ΔB are unaffected by this gap, and the magnetic orbits proceed as two independent copies of the Weyl orbits. For ε <Δ B , the RR ′-mixing can backscatter electrons between segments 2↔3′ and 3↔2′ of the orbits in Fig. 3a , characterized by the length scale . If the distance travelled through the bulk is much less than ℓ M , that is, , then the RR ′-mixing does not typically occur before the electron traverses the bulk. In this case, the mixing is ineffective and the magnetic orbits for each Weyl copy occur essentially independently. On the other hand, if , then, ignoring potential magnetic breakdown effects (see Supplementary Note 4 and Supplementary Fig. 3 ), the electrons penetrate only distance ℓ M into the bulk before returning to the same surface (but switching copies). Then, the orbits occur separately on each surface. The time to traverse such a semiclassical orbit is where the second term accounts for the time virtually spent in the bulk chiral LLs. Applying the semiclassical quantization condition leads to the corresponding energy levels: where we have defined an effective cyclotron mass: The density of states at fixed energy, μ , has periodic-in-1/ B oscillations with period . The behaviour in the intermediate regime, , is shown in Fig. 3e,f . Depending on the relative size of B sat and , the quantum oscillations show re-entrant behaviour ( B sat > B mix , Fig. 3e ) or interference between two oscillations periods ( B sat < B mix , Fig. 3f ). The crossover can be continuously probed in a single sample by varying the field direction. To summarize, by a combination of semiclassical analysis and direct numerical solution, we have demonstrated that up to a critical field strength that is inversely proportional to sample thickness, the surface Fermi arcs of Weyl SMs contribute periodic-in-1/ B quantum oscillations in the density of states. Similar quantum oscillations can occur from arc-like surface states in Dirac SMs. In the Dirac SM case, there are additional complications due to the reduced crystal symmetry of the surfaces and the symmetry-breaking effects of the magnetic field, that interplay with additional symmetry-protected bulk topology. In both cases, density of states oscillations in a field provide experimentally testable fingerprints of the unconventional Fermiology of the Weyl and Dirac surface states. Numerical simulations Numerical simulations were performed by modelling a Weyl SM slab by H = H y + H ⊥ where: and A = Bz ŷ is the vector potential in the Landau gauge corresponding to a uniform magnetic field along ŷ . In this gauge, x momentum is a good quantum number, which just sets the location of the guiding centre for the Landau orbits, and can be taken as zero without loss of generality. Then, we introduce LL raising and lowering operators via: which satisfy canonical commutation relations [ a , a † ]=l. Eigenstates of H y are , with corresponding to eigenvalue ε y = ss ′ υ ⊥ k y . Eigenstates of H ⊥ with eigenvalue ε n were obtained numerically by truncating the oscillator basis a † a | n ›= n | n › to keep a finite number of | n › with n < N max . This truncation breaks the canonical commutation relations of a and a † for states near the cutoff, N max , producing additional spurious low-energy solutions, which are removed by adding a regulator term that energetically penalizes | N max ›. Eigenstates of full Hamiltonian are of the form: where s , s ′=±. Only certain superpositions of such eigenstates will satisfy the boundary conditions at the bottom ( y =0) and top ( y = L ) surfaces of the slab. The proper boundary conditions can be identified by treating the vacuum ( y <0 and y > L ) as an ordinary band-insulator with large gap. Equivalently, we can add a mass term to equation (4) of the form M ( y ) σ z , where M ( y )=0 inside the slab, and M ( y )= M 0 >0 outside the slab. Continuity of the wave functions at the slab boundaries, on taking the limit M 0 →∞, require that Ψ( y =0, L ) be eigenstates of σ x with eigenvalues ±1, respectively. Further details are available in Supplementary Notes 1 and 3 . How to cite this article: Potter, A. C. et al. Quantum oscillations from surface Fermi arcs in Weyl and Dirac semimetals. Nat. Commun. 5:5161 doi: 10.1038/ncomms6161 (2014).